Controlled delivery of bioactive molecules into live cells using the bacterial mechanosensitive channel MscL Bacterial mechanosensitive channels are some of the largest pores in nature. In particular, MscL, with a pore diameter >25 Å, allows passage of large organic ions and small proteins. Functional MscL reconstitution into lipids has been proposed for applications in vesicular-based drug release. Here we show that these channels can be functionally expressed in mammalian cells to afford rapid controlled uptake of membrane-impermeable molecules. We first demonstrate that MscL gating in response to increased membrane tension is preserved in mammalian cell membranes. Molecular delivery is controlled by adopting an established method of MscL charge-induced activation. We then determine pore size limitations using fluorescently labelled model cargoes. Finally, we activate MscL to introduce the cell-impermeable bi-cyclic peptide phalloidin, a specific marker for actin filaments, into cells. We propose that MscL will be a useful tool for gated and controlled delivery of bioactive molecules into cells. Mechanosensitive (MS) ion channels that gate when exposed to mechanical forces are crucial to the perception of sound, touch, gravity or osmotic stress in cells and organisms across all three domains of life [1] , [2] . The first MS channel to be cloned and intensively studied is the large conductance MS channel of Escherichia coli , MscL [3] . MscL opens in response to increased membrane tension; it protects bacteria from membrane damage during high turgor pressure by release of cytoplasmic osmolytes [3] , [4] , [5] , [6] . MscL retains its mechanosensitivity when reconstituted into lipid bilayers, illustrating that activation depends solely on tension in the lipid bilayer [7] . Properties of the lipid environment, such as bilayer thickness, membrane stiffness or spontaneous curvature of the lipid monolayer, affect MscL pressure sensitivity [8] . High-resolution structure of the Myobacterium tubercolosis MscL homologue revealed that it forms a homopentamer of two transmembrane-spanning segment (TM1 and TM2) subunits [9] . The pore is lined primarily by TM1 with a cluster of hydrophobic amino acids constricting the pore [9] , [10] . Opening of the >25 Å diameter pore is accomplished by expansion of both TM1 and TM2 in an iris-like movement. The open channel is non-selective with ~3 nS unitary conductance; it allows the passage of large organic ions and even small proteins down a concentration gradient [3] , [11] , [12] . Previous studies recognized that MscL properties are attractive for potential applications in nanotechnology. MscL can be translated in vitro [13] and functionally reconstituted into lipids, making it ideal for its use in vesicular-based drug release. Moreover, MscL gating underlies a defined mechanism providing a pathway for controlled passage of desired molecules. Substitution of hydrophobic pore residues with cysteine residues and covalent attachment of charged methanethiosulphonate agents was shown to promote MscL gating in the absence of pressure [14] , [15] . This approach enabled the engineering of MscL pores that gate in response to alternative stimuli including light and pH [16] , [17] . MscL may also provide a useful tool in cell biology. Several classes of bioactive molecules that control biological functions or specifically label cellular structures suffer from poor membrane permeability and require physical or chemical methods for efficient delivery. Although cell-penetrating peptides have emerged as valuable tool for translocation of macromolecules across the cell membrane, cargo typically has to be linked to cell-penetrating peptides for efficient uptake [18] . We succeeded in functionally expressing E. coli MS channels in mammalian cells and determined whether MscL could provide a method to control the uptake of small molecules. To our knowledge, this is the first study describing functional expression of E. coli MS channel in mammalian cell lines. We show that the biophysical properties of MscL and MscS in response to increased membrane tension are preserved in mammalian cell membranes. We adopt charge-induced activation [14] , [15] as a method to control MscL gating and delivery of molecules into mammalian cells. Functional expression of the E. coli MS channel MscL was transfected into CHO and HEK-293 cell lines. Excised inside-out patches recorded from MscL, but not vector-transfected cells, display large MS currents in response to increased negative pressure ( Fig. 1a ; Supplementary Fig. S1 ). The threshold of activation was similar in CHO or HEK-293 cells ( Fig. 1b ) and surprisingly consistent with that of MscL recorded from giant spheroplasts or liposomes [3] , [7] . Channels were typically activated when the negative pressure exceeded a threshold in the range of −60 to −120 mm Hg. To account and test for a potential contribution of stress relaxation of the lipid membrane to the MscL activation threshold [19] , we recorded MscL activation under a 1-s linear ramp of pressure, 5 s pulses of gradually increasing pressure, and in response to a series of successively increasing pressure steps ( Fig. 1a ; Supplementary Fig. S1 ). The mean activation threshold was consistent with a minor increase in activation threshold for the 1-s ramp protocol ( Supplementary Fig. S1 ). MscL open probability increased with increasing negative pressure resulting in non-saturating macroscopic currents within the tested pressure range (0–160 mm Hg, Fig. 1a,c ). The pressure required for half-maximal activation ( P 0.5 ), albeit similar in MscL-expressing CHO and HEK-293 cells, was approximately twofold higher ( Fig. 1c , CHO, P 0.5 =160.1±9.0 mm Hg and HEK-293, P 0.5 =147.3±4.3 mm Hg) as compared with MscL recorded from giant spheroplasts or liposomes ( P 0.5 ~75 mm Hg) [7] , [20] , [21] . Previous studies revealed that MscL functional properties are affected by variations in lipid composition [8] , [22] . As such, the difference in lipid membrane composition of mammalian cells and bacteria may at least partly account for the observed discrepancy. The slope conductance of pressure-activated MscL single-channel currents measured in inside–out patches excised from either CHO or HEK-293 cells was, however, consistent with that reported previously for MscL (~2.1 nS, Fig. 1d,e ), given that our recording solution had a ~1.6-fold lower ionic strength as compared with buffers used for spheroplast or liposome recordings [7] , [20] , [21] . 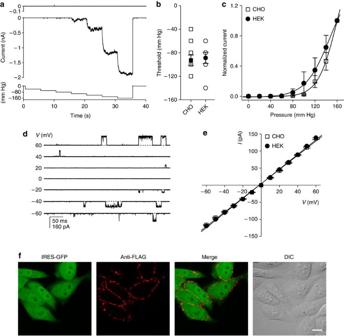Figure 1: Functional expression ofE. coliMscL in mammalian cell lines. (a) Representative currents recorded from excised inside-out patches of vector- (upper panel,n=7) or MscL-transfected (middle panel) CHO cells in response to 5 s pulses of gradually increasing negative pressure (lower panel) atVm=−10 mV. (b) Mean pressure threshold (filled symbols) for MscL is comparable in CHO (−92.7±8.6,n=11) and HEK-293 cells (−88.9±9.5,n=9). Channels were typically activated when the negative pressure exceeded a threshold in the range of −60 to −120 mm Hg. Note: several individual data points (open symbols) have the same value and thus are hidden. (c) Normalized current–pressure relation recorded from inside-out patches of MscL-expressing CHO (n=8) and HEK-293 cells (n=5) atVm=−10 mV. Solid lines represent fits to a Boltzmann equation (CHO,P0.5=160.1±9.0; and HEK-293,P0.5=147.3±4.3). (d) Representative currents recorded from membrane patches of MscL-expressing CHO cells in response to negative pressure (−90 mm Hg) at the indicated voltages. (e) Current–voltage relation of MscL single-channel currents. The conductance was calculated from the slope of the linear regression fits (CHO, 2.08±0.03 nS; and HEK-293, 2.15±0.03 nS). (f) Surface staining of live CHO cells expressing FLAG-tagged MscL in a bicistronic IRES-GFP vector. The FLAG-tag staining is limited to GFP-positive (MscL expressing) cells as illustrated by the differential interference contrast (DIC) image. For panelsb,cande, error bars represent s.e.m. Scale bar, 10 μm. Figure 1: Functional expression of E. coli MscL in mammalian cell lines. ( a ) Representative currents recorded from excised inside-out patches of vector- (upper panel, n =7) or MscL-transfected (middle panel) CHO cells in response to 5 s pulses of gradually increasing negative pressure (lower panel) at V m =−10 mV. ( b ) Mean pressure threshold (filled symbols) for MscL is comparable in CHO (−92.7±8.6, n =11) and HEK-293 cells (−88.9±9.5, n =9). Channels were typically activated when the negative pressure exceeded a threshold in the range of −60 to −120 mm Hg. Note: several individual data points (open symbols) have the same value and thus are hidden. ( c ) Normalized current–pressure relation recorded from inside-out patches of MscL-expressing CHO ( n =8) and HEK-293 cells ( n =5) at V m =−10 mV. Solid lines represent fits to a Boltzmann equation (CHO, P 0.5 =160.1±9.0; and HEK-293, P 0.5 =147.3±4.3). ( d ) Representative currents recorded from membrane patches of MscL-expressing CHO cells in response to negative pressure (−90 mm Hg) at the indicated voltages. ( e ) Current–voltage relation of MscL single-channel currents. The conductance was calculated from the slope of the linear regression fits (CHO, 2.08±0.03 nS; and HEK-293, 2.15±0.03 nS). ( f ) Surface staining of live CHO cells expressing FLAG-tagged MscL in a bicistronic IRES-GFP vector. The FLAG-tag staining is limited to GFP-positive (MscL expressing) cells as illustrated by the differential interference contrast (DIC) image. For panels b , c and e , error bars represent s.e.m. Scale bar, 10 μm. Full size image Further evidence that MscL functional properties are preserved in mammalian cell membranes was derived from experiments that either modulated the transbilayer lateral pressure gradient or changed membrane fluidity [8] , [23] . As such, addition of lysophosphatidylcholine (LPC) to the cytosolic site of a patch strongly favoured MscL transition to the open state, while a change in bath temperature modulated MscL pressure sensitivity ( Supplementary Fig. S2 ). Low temperatures, and thus increased membrane stiffness, resulted in increased pressure sensitivity, while elevated temperatures and increased membrane fluidity decreased MscL pressure sensitivity ( Supplementary Fig. S2 ). Collectively, the results show that MscL is expressed on the surface of mammalian cells, which is further confirmed by expression and live-cell staining of a FLAG-tagged MscL construct ( Fig. 1f ). MscL appeared to localize in clusters on the cell membrane; some protein was also retained in the endoplasmic reticulum ( Fig. 1f ; Supplementary Fig. S1 ). Encouraged by these findings and based on a recent study [24] , we next tested functional expression of E. coli MscS in mammalian cell lines. MscS typically responded when the negative pressure exceeded a threshold of −60 to −100 mm Hg ( Fig. 2a,b ). The mean activation threshold in both CHO and HEK-293 cells (−74±4.3 mm Hg and −80±6.2 mm Hg), as well as the pressure required for half-maximal activation of MscS (88.8±1.1 mm Hg and 84.4±1.3 mm Hg) was, on average, higher than that reported for MscS in spheroplasts or liposomes ( Fig. 2a–c ) [25] , [26] , [27] . Differences in patch geometry, lipid composition and pipette size may contribute to the observed shift. Although it exhibited lower pressure sensitivity in mammalian cell membranes, MscS single-channel conductance was preserved. Depending on the voltage polarity applied, the conductance was between ~380 and ~680 pS, consistent with a ~1.6-fold lower ionic strength of our recording solution ( Fig. 2d,e ). In addition and as reported previously [28] , MscS currents appeared to inactivate in response to prolonged pressure stimuli, indicating that MscS yields a functional MS current with its primary properties preserved in mammalian cell membranes. 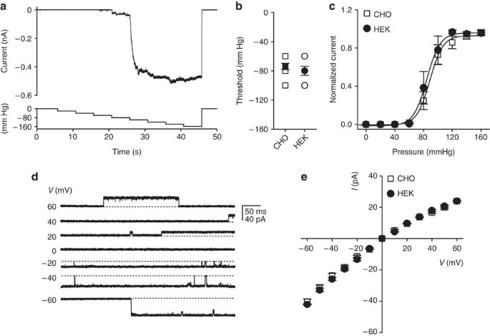Figure 2: Functional expression ofE. coliMscS in mammalian cell lines. (a) Representative current recorded from excised inside-out patches of MscS-transfected (upper panel) CHO cells in response to 5 s pulses of gradually increasing negative pressure (lower panel) atVm=−20 mV. (b) Mean activation threshold (filled symbols) for MscS expressed in CHO (−74±4.3,n=10) and HEK-293 cells (−80±6.2,n=7). Note: several individual data points (open symbols) have the same value and thus are hidden. (c) Normalized current–pressure relation for MscS expressed in CHO (n=10) and HEK-293 cells (n=6) recorded atVm=−20 mV. Solid lines represent fits to a Boltzmann equation (CHO,P0.5=88.8±1.1; and HEK-293,P0.5=84.4±1.3). (d) Representative currents recorded from inside-out patches of CHO cells expressing MscS in response to negative pressure at the indicated voltages. (e) Current–voltage relation of MscS single-channel currents. The conductance was calculated from the slope of linear regression fits (CHO, inward: 652±25.9 pS and outward: 386±15.1 pS; and HEK-293, inward: 685±18.2 pS and outward: 402±18.9 pS). For panelsb,cande, error bars represent s.e.m. Figure 2: Functional expression of E. coli MscS in mammalian cell lines. ( a ) Representative current recorded from excised inside-out patches of MscS-transfected (upper panel) CHO cells in response to 5 s pulses of gradually increasing negative pressure (lower panel) at V m =−20 mV. ( b ) Mean activation threshold (filled symbols) for MscS expressed in CHO (−74±4.3, n =10) and HEK-293 cells (−80±6.2, n =7). Note: several individual data points (open symbols) have the same value and thus are hidden. ( c ) Normalized current–pressure relation for MscS expressed in CHO ( n =10) and HEK-293 cells ( n =6) recorded at V m =−20 mV. Solid lines represent fits to a Boltzmann equation (CHO, P 0.5 =88.8±1.1; and HEK-293, P 0.5 =84.4±1.3). ( d ) Representative currents recorded from inside-out patches of CHO cells expressing MscS in response to negative pressure at the indicated voltages. ( e ) Current–voltage relation of MscS single-channel currents. The conductance was calculated from the slope of linear regression fits (CHO, inward: 652±25.9 pS and outward: 386±15.1 pS; and HEK-293, inward: 685±18.2 pS and outward: 402±18.9 pS). For panels b , c and e , error bars represent s.e.m. Full size image Dye uptake into live cells using MscL Although both channels functionally express in mammalian cells, MscL's larger pore size and potential usefulness in cell biology experiments prompted us to investigate this channel in detail. MscL shares common features with other pore-forming molecules and peptides, creating a pathway for membrane-impermeant molecules. Its large pore diameter (>25 Å) and lack of selectivity [3] , [9] , [10] , [29] are particularly attractive for applications such as drug delivery. While pores often lack defined gating mechanisms, MscL might provide a regulated pathway that permits controlled passage of desired molecules into cells. Previous studies established that charges engineered within the pore of MscL can induce spontaneous channel gating [14] , [15] , [30] . As such, substitution of cysteine for glycine at position 26 (G26C) enables activation of MscL through covalent attachment of charged methanethiosulphonate agents such as MTSET [14] . Utilizing this approach, we confirmed that MTSET (1 mM), applied to the extracellular region of an outside-out patch excised from CHO cells expressing MscL G26C, induces spontaneous channel gating ( Fig. 3a ). Typically, subconducting states and short dwell times were observed before the channel eventually locked into a prolonged open state. Addition of the reducing agent dithiothreitol (DTT, 1 mM) subsequently reversed the effect and facilitated channel closure ( Fig. 3a ). 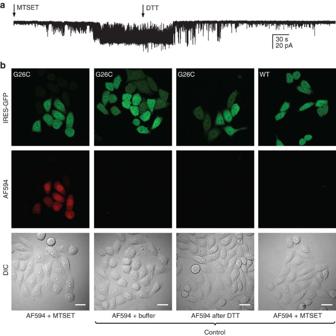Figure 3: Dye delivery through MscL. (a) Outside-out patch recording of MscL G26C. Addition of MTSET (1 mM) to the bath activates MscL G26C while subsequent DTT treatment (1 mM) facilitates channel closure (n=4,Vm=−20 mV). (b) Dye delivery into CHO cells expressing MscL G26C treated for 2 min with MTSET (1 mM) in the presence of 5 μM Alexa Fluor 594 and subsequent exposure for 10 min to DTT (1 mM) to mediate channel inactivation (first column). Dye uptake is limited to GFP-positive (MscL-expressing) cells as illustrated by the differential interference contrast (DIC) image. No delivery was observed under control conditions: incubation with the dye (Alexa Fluor 594, 5 μM, 2 min) in K-aspartate-based delivery solution with no added MTSET (second column); incubation with the dye (Alexa Fluor 594, 5 μM, 2 min) after DTT treatment (1 mM, 10 min) and channel inactivation (third column); in MscL WT-expressing CHO cells treated for 2 min with MTSET (1 mM) in the presence of 5 μM Alexa Fluor 594 (fourth column). AF594, Alexa Fluor 594. Scale bars, 20 μm. Figure 3: Dye delivery through MscL. ( a ) Outside-out patch recording of MscL G26C. Addition of MTSET (1 mM) to the bath activates MscL G26C while subsequent DTT treatment (1 mM) facilitates channel closure ( n =4, V m =−20 mV). ( b ) Dye delivery into CHO cells expressing MscL G26C treated for 2 min with MTSET (1 mM) in the presence of 5 μM Alexa Fluor 594 and subsequent exposure for 10 min to DTT (1 mM) to mediate channel inactivation (first column). Dye uptake is limited to GFP-positive (MscL-expressing) cells as illustrated by the differential interference contrast (DIC) image. No delivery was observed under control conditions: incubation with the dye (Alexa Fluor 594, 5 μM, 2 min) in K-aspartate-based delivery solution with no added MTSET (second column); incubation with the dye (Alexa Fluor 594, 5 μM, 2 min) after DTT treatment (1 mM, 10 min) and channel inactivation (third column); in MscL WT-expressing CHO cells treated for 2 min with MTSET (1 mM) in the presence of 5 μM Alexa Fluor 594 (fourth column). AF594, Alexa Fluor 594. Scale bars, 20 μm. Full size image To test whether MscL G26C enables controlled delivery of molecules into cells, we first monitored uptake of an Alexa dye through the pore of MscL. Cells were treated for 2 min with MTSET in the presence of Alexa Fluor 594 (5 μM) to modify MscL G26C and trigger dye uptake, and then incubated with DTT (10 min) to induce channel closure. Only cells expressing MscL G26C, as monitored by green fluorescence (the construct being expressed from a bicistronic IRES-green fluorescent protein (GFP) vector), but not surrounding cells, showed significant dye uptake ( Fig. 3b ). No delivery was observed in MscL G26C-expressing cells in the absence of MTSET or after inactivation with DTT ( Fig. 3b ), excluding endocytosis as a mechanism for dye uptake and confirming successful channel closure following DTT treatment. Accordingly, CHO cells expressing wild-type MscL, which lacks endogenous cysteine residues and is therefore immune to covalent modification by methanethiosulphonate agents, did not exhibit dye uptake after MTSET treatment ( Fig. 3b ). We next examined MscL-mediated dye delivery in several standard mammalian cell lines (HEK-293, HeLa and COS-7). All tested cell lines expressed MscL G26C; MTSET triggered activation of the channel as monitored by Alexa Fluor 594 (5 μM) uptake ( Supplementary Fig. S3 ). The data demonstrate that charge-induced activation of MscL G26C is a useful method to deliver ~700 Da molecules into mammalian cells. Cell viability after MscL activation The large pore size of MscL is attractive for its use as a potential delivery tool, but at the same time its >25 Å diameter and large conductance [3] , [9] , [10] , [29] may cause cytotoxic effects. To identify an effective open time of MscL that could be used for delivery of molecules without inducing cell death, we established a CHO cell line stably expressing MscL G26C (hereafter referred to as CHO-MscL-G26C) and screened for uniform dye uptake ( Fig. 4a ; Supplementary Fig. S4 ). Cytotoxicity of MscL activation was assessed by the use of a cell proliferation assay (MTT assay). CHO cells stably expressing the wild-type channel (hereafter referred to as CHO-MscL-WT) served as control ( Fig. 4 ; Supplementary Fig. S4 ). Cells were exposed to MTSET for different durations ranging from 30 s to 20 min followed by a 10-min treatment with DTT, repetitive washing steps and incubation in growth media for 24 h before being assayed for cell viability. MscL activation for up to 8 min was not toxic in a K-aspartate-based buffer (Methods). However, at times longer than 10 min, MTSET treatment significantly decreased cell viability of CHO-MscL-G26C cells; covalent modification of endogenous cysteine residues exposed on the cell surface of CHO-MscL-WT cells did not induce cytotoxicity. At 10- and 20-min exposure times, viability of CHO-MscL-G26C cells was 42.2% and 9.1%, respectively, setting the upper limit for safe delivery of molecules to live cells in K-aspartate buffer to 8 min ( Fig. 4b ). In a standard extracellular solution (Ringer solution), cell viability was significantly decreased after 4-min MTSET exposure ( Supplementary Fig. S4 ). 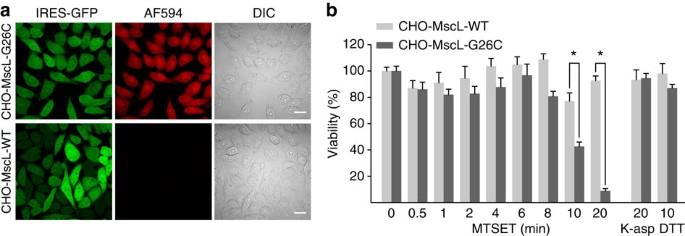Figure 4: Cell viability and integrity after MscL activation by MTSET. (a) Efficient delivery of 10 μM Alexa Fluor 594 into stable CHO-MscL-G26C cells treated for 2 min with MTSET (1 mM) in the presence of the dye (upper row). The control polyclonal CHO-MscL-WT cell line did not take up dye (lower row). AF594, Alexa Fluor 594; DIC, differential interference contrast. Scale bars, 20 μm. (b) Cell viability as a function of MscL activation time. The monoclonal CHO-MscL-G26C cell line and the polyclonal CHO-MscL-WT cell line (serving as a control) were treated for the indicated time with MTSET (1 mM) followed by DTT exposure (1 mM, 10 min) to facilitate MscL inactivation. To control for nonspecific effects of the delivery solution or the reducing agent, both cell lines were incubated for 20 min in the K-aspartate (K-asp)-based delivery solution and for 10 min with DTT (1 mM). Viability was assessed using a MTT assay. Data were collected at three independent times in quadruplicate. Error bars represent s.e.m.;P=0.0094 (CHO-MscL-G26C versus CHO-MscL-WT control after 10 min MTSET treatment) andP<0.001 (CHO-MscL-G26C versus CHO-MscL-WT control after 20 min MTSET treatment; Student's unpairedt-test). Figure 4: Cell viability and integrity after MscL activation by MTSET. ( a ) Efficient delivery of 10 μM Alexa Fluor 594 into stable CHO-MscL-G26C cells treated for 2 min with MTSET (1 mM) in the presence of the dye (upper row). The control polyclonal CHO-MscL-WT cell line did not take up dye (lower row). AF594, Alexa Fluor 594; DIC, differential interference contrast. Scale bars, 20 μm. ( b ) Cell viability as a function of MscL activation time. The monoclonal CHO-MscL-G26C cell line and the polyclonal CHO-MscL-WT cell line (serving as a control) were treated for the indicated time with MTSET (1 mM) followed by DTT exposure (1 mM, 10 min) to facilitate MscL inactivation. To control for nonspecific effects of the delivery solution or the reducing agent, both cell lines were incubated for 20 min in the K-aspartate (K-asp)-based delivery solution and for 10 min with DTT (1 mM). Viability was assessed using a MTT assay. Data were collected at three independent times in quadruplicate. Error bars represent s.e.m. ; P =0.0094 (CHO-MscL-G26C versus CHO-MscL-WT control after 10 min MTSET treatment) and P <0.001 (CHO-MscL-G26C versus CHO-MscL-WT control after 20 min MTSET treatment; Student's unpaired t -test). Full size image Delivery efficiency and size limitations To characterize MscL-mediated delivery of molecules to live cells, we chose fluorescent dyes (Alexa Fluor 594, ~760 Da), and 3,000- and 10,000-Da Texas Red dextran conjugates as model cargoes. Delivery efficiency visibly increased with activation time (that is, incubation with MTSET for 30 s versus 8 min) and decreased with increased molecular weight or molecule size ( Fig. 5a,b ). While molecules < 1,000 Da (that is, Alexa Fluor 594) readily accumulated in CHO-MscL-G26C cells after short activation times, passage of larger molecules (3,000 and 10,000 Da) required extended activation times ( Fig. 5a,b ). The upper size limit for molecules that can diffuse through MscL under the conditions tested was ≤10,000 Da, which is consistent with previously reported size limits [11] , [12] . Analysing the average pixel intensity in cells per field revealed little effective delivery of the 10,000-Da Texas Red dextran even after prolonged MscL activation ( Fig. 5b ). No uptake into CHO-MscL-G26C cells was observed for any of the model cargoes at 8-min incubation time in the absence of MTSET. A few cells showed weak fluorescence after DTT treatment and subsequent incubation with Alexa Fluor 594, suggesting incomplete breaking of disulphide bonds and incomplete channel closure after extended MTSET exposure time (8 min) ( Supplementary Fig. S5 ). 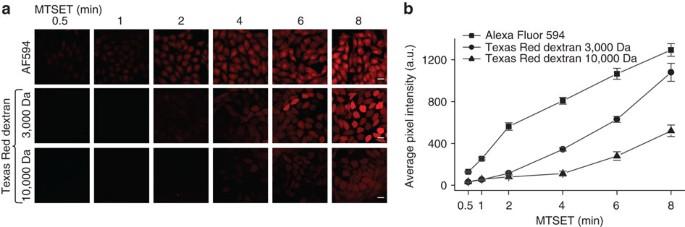Figure 5: Activation time and molecular weight control delivery efficiency through MscL. (a) Live-cell fluorescence imaging of MscL-mediated dye (Alexa Fluor 594, ~760 Da, 20 μM) or dextran–dye conjugate (Texas Red dextran 3,000 and 10,000 Da, 100 μM) delivery using the monoclonal CHO-MscL-G26C cell line. The delivery efficiency increases with increased activation time (incubation with MTSET, 1 mM) and decreases with increased molecule size/molecular weight. Note: 3,000 and 10,000 Da dextran preparations contain branched polymers with molecular weights in the range of 1,500–3,000 and 9,000–11,000 Da, respectively. AF594, Alexa Fluor 594. Scale bars, 20 μm. (b) Average pixel intensity in cells per field (displaying dye or dextran–dye conjugate delivery) as a function of MscL G26C activation time. The mean fluorescent intensity at each time point was calculated for five independent fields. Error bars represent s.e.m. Figure 5: Activation time and molecular weight control delivery efficiency through MscL. ( a ) Live-cell fluorescence imaging of MscL-mediated dye (Alexa Fluor 594, ~760 Da, 20 μM) or dextran–dye conjugate (Texas Red dextran 3,000 and 10,000 Da, 100 μM) delivery using the monoclonal CHO-MscL-G26C cell line. The delivery efficiency increases with increased activation time (incubation with MTSET, 1 mM) and decreases with increased molecule size/molecular weight. Note: 3,000 and 10,000 Da dextran preparations contain branched polymers with molecular weights in the range of 1,500–3,000 and 9,000–11,000 Da, respectively. AF594, Alexa Fluor 594. Scale bars, 20 μm. ( b ) Average pixel intensity in cells per field (displaying dye or dextran–dye conjugate delivery) as a function of MscL G26C activation time. The mean fluorescent intensity at each time point was calculated for five independent fields. Error bars represent s.e.m. Full size image Controlled cellular uptake of phalloidin MscL has been shown to allow release of solutes from E. coli during hypoosmotic shock [4] , [5] . At high turgor pressure, MscL activation may permit protein efflux as demonstrated recently by dual-colour fluorescence burst analysis [12] . Small proteins up to ~6,500 Da passed through MscL. Several small proteins or peptides can act as substrates, inhibitors or modulators of biological functions, but typically possess poor membrane permeability and often require molecular vehicles to gain access to the cell's cytosolic compartments. One such example is the cell-impermeable bi-cyclic peptide phalloidin, a toxin from Amanita phalloides , commonly used as a specific marker for actin filaments. Until recently, delivery of phalloidin was limited to permeabilized cells or required microinjection. Reshetnyak et al . [31] showed effective translocation of phalloidin using a synthesized conjugate of a pH-responsive insertion peptide (pHLIP) and fluorescent phalloidin. To assess whether phalloidin could pass through MscL and stain actin filaments in live cells, we stimulated CHO-MscL-G26C cells with MTSET in the presence of an Alexa Fluor 568 phalloidin conjugate (~1,600 Da). We observed a staining pattern characteristic of actin filaments that was absent in control cells treated with DTT before incubation with the phalloidin–dye conjugate ( Fig. 6 ). As a control, CHO-MscL-WT cells incubated for the same duration with MTSET in the presence of the phalloidin–dye conjugate were not labelled by phalloidin ( Fig. 6 ). 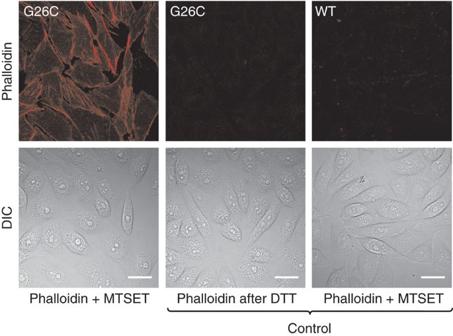Figure 6: MscL-mediated delivery of phalloidin. Fluorescence images of CHO-MscL-G26C cells activated for 4 min with MTSET (1 mM) in the presence of 400 nM Alexa Fluor 568 phalloidin (left column) or in control delivery experiments adding phalloidin (4 min) only after inactivation of MscL G26C by DTT (1 mM, 10 min, middle column) or to CHO-MscL-WT cells in the presence of MTSET (4 min, right column). Bright staining of actin filaments was observed after MscL-mediated delivery of phalloidin, but not in control delivery experiments. DIC, differential interference contrast. Scale bars, 20 μm. Figure 6: MscL-mediated delivery of phalloidin. Fluorescence images of CHO-MscL-G26C cells activated for 4 min with MTSET (1 mM) in the presence of 400 nM Alexa Fluor 568 phalloidin (left column) or in control delivery experiments adding phalloidin (4 min) only after inactivation of MscL G26C by DTT (1 mM, 10 min, middle column) or to CHO-MscL-WT cells in the presence of MTSET (4 min, right column). Bright staining of actin filaments was observed after MscL-mediated delivery of phalloidin, but not in control delivery experiments. DIC, differential interference contrast. Scale bars, 20 μm. Full size image For the past two decades, MscL has served as a model molecule for MS channels. Functional reconstitution of MscL into liposomes provided insight into the interplay between lipid bilayer mechanical properties and protein structure and function [8] , [21] , [22] , [32] . Here, we report functional expression of E. coli MS channel in mammalian cell lines and present evidence that MscL constitutes a useful tool for controlled delivery of molecules to live cells. Consistent with its function as pressure valve in bacteria [4] , [5] , we show that increased membrane tension activates MscL in excised patches of mammalian cell membranes. MscL properties were preserved in both cell lines tested (CHO and HEK-293), and live-cell staining of a FLAG-tagged construct confirmed its membrane localization. Our finding that MscS also functionally expresses in mammalian cell lines may facilitate analysis of bacterial MS channels and complement existing techniques [3] , [7] , [13] , [24] , [33] . MscL combines two intriguing features for biotechnology applications; first, the large pore (>25 Å) and lack of selectivity [3] , [9] , [10] , [29] promotes passage of both ionic and non-ionic molecules, and second, intrinsic and modulated channel gating provides a defined control mechanism for passage of desired molecules. As such, MscL has been applied as a controllable nanovalve in vesicular-release devices, and molecular dynamic simulations provided further mechanistical inside into the release of content from pressurized liposomes [16] , [17] , [34] . Previous studies typically relied on thiol-reactive compounds to accomplish vesicular release [14] , [15] , [16] , [17] . Adopting this method, we employed MscL for a controllable delivery device with potential applications in cell biology. Using MTSET and DTT to control gating of a genetically engineered MscL channel (G26C), we illustrate successful uptake of model cargo, including Alexa Fluor 594 and Texas Red dextran, into mammalian cells. Consistent with previous reports, we show that molecules ≤ 3,000 Da rapidly accumulate in CHO cells, while the larger 10,000-Da Texas Red dextran barely passed through the channel pore. A lower diffusion rate may account for much of the decreased delivery efficiency of larger cargo through MscL. Another limiting factor may include the channel's preference for subconducting states at short MTSET incubation times and consequently a narrower pore [14] . The exact geometric and charge limitations of cargo that MscL can translocate remain to be studied. A recent study showed that MscL G26C treated with either positively or negatively charged methanethiosulphonate agents has ion selectivity that differs from the wild-type channel [35] . Future studies will examine how different charges engineered within the pore of MscL G26C may influence the permeation of charged molecules. Our data suggest that larger molecules require extended MscL activation time for efficient delivery, which in turn increases cytotoxicity. Cytotoxicity induced by the prolonged activation of MscL might be reduced using the recently engineered smaller-pore MscL channel [36] . Alternatively, MscL proteins with different pore sizes may provide increased versatility for applications in cell biology. Although neither MTSET nor DTT affected cell proliferation, we cannot exclude acute perturbation of cellular signalling evoked by covalent modification of endogenous cysteine residues. While light and pH have been reported to trigger activation of engineered MscL proteins, both approaches are based on covalent modification of thiol groups [16] , [17] . Our finding that MscL mediates rapid and minimally disruptive uptake of fluorescently labelled phalloidin provides an appealing alternative method for live-cell visualization of the distribution of F-actin within cells. The ability of MscL to deliver a bi-cyclic peptide to mammalian cells additionally holds promise for the use of MscL as a tool for peptide and/or macromolecule delivery. Bioactive peptides are often used as pharmacological tools, and can function as ligand for transcription factors and cellular receptors or exhibit immunosuppressive properties. Although it remains to be tested, MscL may provide a platform to assess peptide activity within cells and screen for new peptide drugs. Thus, MscL constitutes a new tool with potential future applications for transport and delivery, acute cell permeabilization or even induced cell death. Finally, functional expression of bacterial MS channel in mammalian cell membranes might prove useful when employed as tools to probe membrane tension in living cells. cDNA constructs The E. coli MscL and MscS coding sequences were a generous gift from Boris Martinac (Victor Chang Cardiac Research Institute, Australia). Both cDNAs were subcloned into pIRES2-eGFP (Clontech). The MscL-FLAG construct in pIRES2-eGFP was made by insertion of the FLAG-tag sequence (DYKDDDDK) after position I68 of E. coli MscL. MscL G26C mutagenesis was performed using overlap-extension PCR with synthetic complementary oligonucleotides. All cDNA constructs were verified by DNA sequencing. Cell lines and transfection CHO, HEK-293, HeLa and COS-7 cells were transfected using Lipofectamine 2000 (Invitrogen), plated onto glass cover slips, and used for electrophysiological recordings and/or delivery experiments 18–48 h after transfection. CHO cells stably expressing the E. coli MscL wild-type construct (CHO-MscL-WT) or MscL G26C (CHO-MscL-G26C) in pIRES2-eGFP were obtained after transfection with the respective cDNA, selection of stable cells with G-418 (Invitrogen) and further selection by fluorescence-activated cell sorting of GFP-positive cells. To obtain a monoclonal MscL G26C CHO cell line, fluorescence-activated cell sorting-sorted cells were diluted and selected in 96-well plates for single colony growth. Colonies were subsequently picked and screened for uniform dye uptake. Electrophysiology The channel activities of recombinantly expressed E. coli MscL and MscS were examined in excised patch recordings in symmetric potassium (in mM; 150 KCl, 20 HEPES, 1 EGTA, pH 7.4). The bath solution in outside-out patch recordings was equivalent to the solution used for delivery experiments (in mM; 140 KOH, 100 aspartate, 12 NaOH, 4 HCl, 1 MgCl 2 , 2 Mg-ATP, 10 HEPES, pH 7.3). Electrodes with a resistance of 1.5–2.5 MΩ and a pipette bubble number of 5.5–6.5 (ref. 37 ) were pulled from borosilicate glass (WPI) using a Flaming/Brown pipette puller (Sutter Instruments). Pressure steps and ramps were applied using a HSPC-1 high-speed pressure system (ALA Scientific) [38] controlled by pClamp software (Molecular Devices). A P-V pump unit was used as a pressure/vacuum source (ALA Scientific). Bath temperature was regulated using a bipolar temperature controller and an in-line heater/cooler with continuous perfusion (Warner Instruments). The bath temperature was monitored using a thermistor placed in close proximity to the recording electrode. Membrane voltage was controlled and currents recorded using an Axopatch 200B amplifier (Molecular Devices). All recordings were low-pass filtered at 5 kHz, and acquired at 10 or 20 kHz. Data analysis was performed off-line using Clampfit 9 (Molecular Devices) and Origin 7 (OriginLab), and currents further digitally filtered off-line for display purposes. Data are presented as mean±s.e.m. Statistical comparison was made using Student's unpaired t -test ( P -value <0.05 was considered statistically significant). The normalized current–pressure relation for MscL and MscS was fitted to a Boltzmann function ( I = I max +( I min − I max )/(1+exp (( P – P 0.5 )/ k )), where I max and I min are the maximum and minimum current values, P is the test pressure, P 0.5 is the pressure activation midpoint and k is the slope factor). Single-channel conductance was calculated from the slope of linear regression fits and the open probability (NP OPEN ) after LPC treatment was computed by the equation NP OPEN = T OPEN /( T OPEN + T CLOSED ) using Clampfit 9 (Molecular Devices). Immunofluorescence staining For live-cell staining of CHO cells transfected with the MscL-FLAG construct, cells were incubated for 30 min at 4 °C with monoclonal anti-FLAG M2 IgG (2 μg ml −1 , Sigma). Nonspecific binding was blocked by the addition of 2% goat serum and 2% BSA (Sigma). Cells were washed 3× in blocking buffer followed by incubation for 30 min at room temperature (RT) with an Alexa Fluor 546-conjugated anti-mouse IgG secondary antibody (2 μg ml −1 , Invitrogen). For staining of fixed cells (4% paraformaldehyde, 45 min, RT), MscL-FLAG-transfected cells were incubated in 0.1% Triton X-100 in PBS for 45 min at RT and nonspecific binding blocked by subsequent incubation in 2% goat serum and 2% BSA for 45 min at RT. Labelling was carried out by incubation with anti-FLAG IgG (2 μg ml −1 , 1 h, RT) followed by anti-mouse IgG secondary antibody (2 μg ml −1 , 30 min, RT). Images were acquired with a FluoView-1000 laser scanning confocal microscope (Olympus). Delivery experiments In a typical delivery experiment, stably or transiently transfected cells were plated on glass cover slips 24–48 h before the experiment. After removal from the 37 °C, 5% CO 2 incubator, cover slips were placed in Ringer solution (in mM; 145 NaCl, 5 KCl, 2 CaCl 2 , 1 MgCl 2 , 10 HEPES, 10 glucose, pH 7.4) and kept at RT for the entire length of the experiment. The cells grown on a cover slip were first briefly rinsed in the K-aspartate-based delivery solution (in mM; 140 KOH, 100 aspartate, 12 NaOH, 4 HCl, 1 MgCl 2 , 2 Mg-ATP, 10 HEPES, pH 7.3) and subsequently incubated with MTSET (1 mM) to activate MscL G26C and allow for delivery of the desired molecule. Channel closure was achieved after a brief rinse in K-aspartate-based solution by incubation with DTT (1 mM) for 10 min. MTSET was diluted from a 10 mM stock, which was freshly prepared before each use and kept on ice. After delivery of the respective molecule (dye, dye–dextran conjugate, phalloidin), cover slips were transferred to a live imaging chamber in Ringer solution and imaged by laser scanning fluorescence confocal microscopy (Fluoview-1000, Olympus). Confocal images were analysed using Image-J software (NIH). The delivery efficiency of different size molecules at discrete MscL activation times was measured by analysing the average pixel intensity in cells per field. First, images were background-subtracted. For each field of view analysed, a mask of the areas corresponding to cells expressing MscL was created by thresholding of the GFP channel (the construct being expressed from a bicistronic IRES-GFP vector). This mask was subsequently applied to the fluorescence image of the delivered molecule (typically a Texas Red or Alexa Fluor 594 conjugate), followed by calculation of the mean fluorescence pixel intensity. The mean fluorescence intensity within cells for the whole field was calculated for five independent fields of view and averaged. To avoid detector saturation, acquisition parameters (for example, PMT voltage and confocal aperture) were established first for the conditions giving maximum dye fluorescence (that is, 8 min activation) and kept constant across all experiments. MTT assay The metabolic integrity of cells after activation of E. coli MscL for different durations was assessed using MTT following the manufacturer's instructions (Cayman Chemical). Briefly, cells were seeded at 0.5×10 5 ml −1 per well in 96-well plates and cultured in a CO 2 incubator at 37 °C for 24 h. Following the typical delivery protocol, cells were treated for different durations with MTSET (0–20 min) to induce channel opening in MscL G26C-expressing cells, but not MscL WT-expressing control cells. To further control for side effects of the delivery solution or the reducing agent, both cell lines were treated with DTT alone (1 mM, 10 min) or incubated in the K-aspartate-based delivery solution for 20 min followed by a 10-min DTT treatment. Cells were subsequently placed in fresh growth media (DMEM/F12), and incubated at 37 °C, 5% CO 2 for 24 h. MTT absorbance was measured using a microplate reader (PerkinElmer). Cell survival data were collected 2–3 independent times in quadruplicate, background subtracted and normalized to untreated control cells. Chemicals MTSET was purchased from Toronto Research Chemicals, DTT and LPC from Sigma, and Alexa Fluor 594 hydrazide, Texas Red dextran (3,000 and 10,000 Da) and Alexa Fluor 568 phalloidin were obtained from Invitrogen. J.F.D. and D.E.C. designed the research; J.F.D. performed the experiments and analysed the data; S.F. contributed to the research design and analysis; and J.F.D., S.F. and D.E.C. wrote the paper. How to cite this article: Doerner J. F. et al . Controlled delivery of bioactive molecules into live cells using the bacterial mechanosensitive channel MscL. Nat. Commun. 3:990 doi: 10.1038/ncomms1999 (2012).